Manipulation and coherence of ultra-cold atoms on a superconducting atom chip The coherence of quantum systems is crucial to quantum information processing. Although superconducting qubits can process quantum information at microelectronics rates, it remains a challenge to preserve the coherence and therefore the quantum character of the information in these systems. An alternative is to share the tasks between different quantum platforms, for example, cold atoms storing the quantum information processed by superconducting circuits. Here we characterize the coherence of superposition states of 87 Rb atoms magnetically trapped on a superconducting atom chip. We load atoms into a persistent-current trap engineered next to a coplanar microwave resonator structure, and observe that the coherence of hyperfine ground states is preserved for several seconds. We show that large ensembles of a million of thermal atoms below 350 nK temperature and pure Bose–Einstein condensates with 3.5 × 10 5 atoms can be prepared and manipulated at the superconducting interface. This opens the path towards the rich dynamics of strong collective coupling regimes. The quantum physics of interfaces is attracting great interest because quantum state transfer between subsystems is required for quantum measurements, quantum information processing and quantum communication [1] . To overcome the fast decoherence of superconducting qubits, the engineering of various hybrid quantum systems recently became a subject of intensive research [2] , [3] , [4] , [5] , [6] , [7] , [8] . The success of strong coupling between superconducting two-level systems and microwave cavities [9] , the implementation of quantum algorithms with superconducting circuits [10] , [11] , [12] and the successful realization of superconducting surface traps for ultra-cold atoms [13] , [14] , [15] encourage the development of superconductor/cold atom hybrids. So far, some fundamental interactions between the two systems have been observed [15] , [16] , [17] . However, coherent coupling between the systems remains a scientific and technological challenge. Although theoretical proposals suggest using atomic ensembles as quantum memories in a hybrid quantum computer [18] , [19] , [20] , the trapping of atoms in the vicinity of a superconducting coplanar microwave resonator (CPR) is still required. Long coherence times and state transfer are central issues for quantum information processing. In cold atomic ensembles, the fine control of inhomogeneous dephasing sources [21] , [22] allows long storage times of a single collective excitation [23] . A similar control in chip-based trapped atomic clocks [24] allowed to preserve coherent states of rubidium hyperfine levels over tens of seconds [25] . In addition, the energy spectrum of rubidium atoms can be used to convert the quantum information to the near infrared, in the telecom band [22] , where long-distance quantum communication can be realized [26] . Hybrid systems of cold atoms and superconductors are therefore very appealing for a solid state, atomic and photonic quantum interface. Nevertheless, the question how to preserve such coherence and optical properties in the complex environment of a hybrid system needs to be solved. Here, we report on the preparation of coherent atomic samples at a superconducting interface. We load ultra-cold 87 Rb atoms into a magnetic trap generated by a superconducting niobium thin film structure. We measure exceptionally long lifetimes of fully spin-polarized states (>4 min). In either of the hyperfine ground states of rubidium, we reach the critical temperature of Bose−Einstein condensation with more than one million atoms. The coherence of the superpositions of these ground states is measured for various positions on the superconducting interface. In a self-centred persistent-current trap engineered in the vicinity of a CPR we observe a coherence time T 2 ~8 s. This demonstrates that cold atom trap inhomogeneities can be controlled in this complex environment to a metrological level, paving the way towards long-living single excitations. Experimental apparatus The experimental apparatus combines a cryostat (Janis ST-400, 2 W cooling power) holding a superconducting atom chip and a cold atom setup integrated in a single ultrahigh vacuum chamber ( Fig. 1a ). The pressure of the chamber, as measured by an ion gauge, is ~10 −11 mbar. Owing to the strong cryopumping, the pressure close to the chip surface is probably even lower. Such vacuum constitutes an excellent heat isolation between the superconducting chip surface at a temperature of T =4.2 and the room temperature electromagnets that are used for the preparation of cold atomic samples [27] . A copper radiation shield at ~20 K protects the chip from the room temperature thermal radiation. A slit of 2 mm height on the shield gives optical access to an optical tweezers that transports atom clouds from the room temperature environment to the superconducting atom chip. 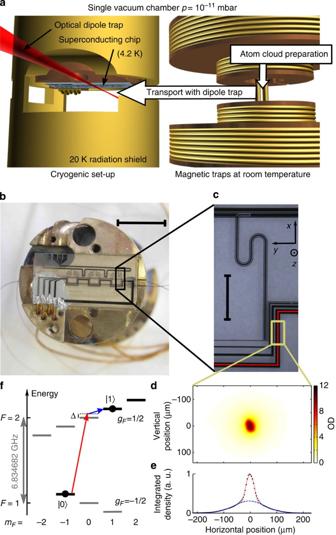Figure 1: Hybrid system of ultra-cold atoms and superconductors. (a)In-vacuosetup (to scale): on the right side, the atoms are trapped and cooled in a room temperature environment. The left part shows the superconducting chip attached to the cryostat at 4.2 K and surrounded by a gold-plated radiation shield at ~20 K. The atoms are transported from one environment to the other (40 mm distance) by optical tweezers. (b) Photograph of the superconducting atom chip mounted onto an oxygen-free copper holder. Scale bar, 1 cm. (c) Microscope image of the superconducting trapping structure. Visible are fourZ-wires for trapping, one being highlighted by the red line and a quarter-wave CPR capacitively coupled to the feedline. Scale bar, 1 mm. (d) Absorption image of a BEC in state |0withNBEC=3 × 105atoms after 15 ms TOF. Colour scale corresponds to optical density (OD). (e) Normalized integrated density showing the bi-modal structure of a BEC (black points). In dashed blue is shown a fit to the thermal background and in dotted red a fit to the central Thomas Fermi profile. (f) Energy diagram of87Rb in a magnetic field. In dark are shown the three magnetically trappable states. The coupling of |F=1,mF=−1(|0) and |F=2,mF=1(|1) is realized by a two-photon transition. Figure 1: Hybrid system of ultra-cold atoms and superconductors. ( a ) In-vacuo setup (to scale): on the right side, the atoms are trapped and cooled in a room temperature environment. The left part shows the superconducting chip attached to the cryostat at 4.2 K and surrounded by a gold-plated radiation shield at ~20 K. The atoms are transported from one environment to the other (40 mm distance) by optical tweezers. ( b ) Photograph of the superconducting atom chip mounted onto an oxygen-free copper holder. Scale bar, 1 cm. ( c ) Microscope image of the superconducting trapping structure. Visible are four Z -wires for trapping, one being highlighted by the red line and a quarter-wave CPR capacitively coupled to the feedline. Scale bar, 1 mm. ( d ) Absorption image of a BEC in state |0 with N BEC =3 × 10 5 atoms after 15 ms TOF. Colour scale corresponds to optical density (OD). ( e ) Normalized integrated density showing the bi-modal structure of a BEC (black points). In dashed blue is shown a fit to the thermal background and in dotted red a fit to the central Thomas Fermi profile. ( f ) Energy diagram of 87 Rb in a magnetic field. In dark are shown the three magnetically trappable states. The coupling of | F =1, m F =−1 (|0 ) and | F =2, m F =1 (|1 ) is realized by a two-photon transition. Full size image The superconducting chip with Z -shaped wires (red line) and a quarter-wave CPR structure is shown in Fig. 1b,c . The niobium film structures (500 nm thickness) were fabricated on monocrystalline sapphire by magnetron sputtering, optical lithography and reactive ion etching (SF 6 ). Niobium is, in our experimental conditions, a type II superconductor with a transition temperature of 9.2 K. At 4.2 K, the wires carry mean current densities of up to 4 × 10 6 A cm −2 , corresponding to a current of 1 A for a wire of 50 μm width. Supply wires (normal conducting copper) are connected by ultrasonic soldering to the niobium. The sapphire substrate is similarly soldered to the copper mount of the cryostat. Two superconducting wires of 100 μm diameter pass below the chip and help to maintain the longitudinal confinement of the trap ( Fig. 1b ). The preparation of atomic clouds follows the standard techniques of magneto-optical (MOT) and magnetic trapping (see Methods for details) and leads, in the room temperature environment, to a cold cloud of 5 × 10 6 atoms at T <1.5 μK. After transfer to an optical dipole trap, the cloud is transported into the cryogenic environment to the loading position at ~400 μm from the superconducting chip surface. The atoms are then transferred into a harmonic magnetic trap [28] formed by superposing the field generated by the current I Trap =0.8 A driven through the largest Z -shaped trapping wire with a homogeneous magnetic bias field B bias =4 G applied along y and a magnetic offset field B off =0.6 G applied along x . The atoms loaded are then adiabatically compressed in a trap with oscillation frequencies { ω x , ω y , ω z }/2 π ={19,145,128} Hz and subsequently cooled by radio-frequency (RF) forced evaporation to temperatures of ~200 nK. By changing the length of the initial MOT phase (1–10 s), the atom number in the superconducting trap (10 4 –10 6 ) and the final state (thermal cloud or Bose−Einstein condensate (BEC)) can be conveniently controlled without affecting the temperature. Owing to the strong cryopumping and the suppression of thermally driven magnetic field fluctuations [17] , the lifetimes of the atoms in such a surface trap are predicted to be exceptionally long [29] , [30] , [31] . For a cloud of N at =10 5 atoms polarized in state | F =1, m F =−1 ( Fig. 1f ) at a density of 10 13 at cm −3 held in the compressed trap with an offset field B off =0.6 G, we measure a lifetime of more than 4 min. From this result and the lifetime of 10 min obtained in Emmert et al. [32] , we expect excellent vacuum conditions for sub-kelvin cryostats where both cold atoms and superconducting circuits will behave quantum mechanically. We form pure BECs with up to 3.5 × 10 5 atoms in either of the spin states, | F =1, m F =−1 or | F =2, m F =2 . The lifetime of such a condensate in the | F =1, m F =−1 state in a trap with frequencies {15, 72, 43} Hz is 30(3) s and is density limited by three-body collisional losses [33] . Such high atom number BECs are of special interest for superradiance experiments, for the realization of an on-chip maser [34] and for quantum information protocols in which an effective strong coupling regime is reached by a collective enhancement [20] . For the latter a BEC is not mandatory. It could be better positioned than a thermal cloud but would suffer from a lower atom number and related weaker collective enhancement. In the following, we explore the properties of the cold cloud in the vicinity of the superconducting CPR. We first consider the positioning of atoms in the close vicinity of the CPR, where we additionally engineer a persistent-current trap. As a further step, we study the coherence of atomic superposition states in different positions of the CPR mode volume. The resonator used in this report is designed to be 250 MHz off resonance from any hyperfine transitions and should therefore not affect the internal state dynamics of the atoms. Positioning of atomic clouds into a CPR In a CPR, the electromagnetic fields are concentrated in the gaps between the ground planes and the central conductor. To maximize the atom–cavity coupling, atoms need to be positioned in the close vicinity of these gaps. Nevertheless, for trap-wire distances smaller than the wire width, the trapping parameters are significantly affected by the Meissner–Ochsenfeld effect (MOE) [16] , [36] . To limit such deformations in the vicinity of the CPR, the design shown in Fig. 1c includes four Z -shaped wires with widths ranging from 100 to 15 μm. Starting from the largest Z -wire trap, the atoms are first horizontally transferred to the third Z -wire trap. The fourth and last wire (15 μm width) revealed to be unnecessary. At 100 μm below the third trapping wire, the trap needs to be rotated towards the CPR gap. Two parameters are classically used to manipulate the atoms on a chip; the value of the trapping wire current modifies the trap-wire distance and the direction of the bias field rotates the trap around the trapping wire. Because of the MOE, positioning that is straightforward for a normal conducting chip is more subtle for a superconducting atom chip. In the present case, we take advantage of the conservation of magnetic flux in superconducting loops to directly guide the atoms below the gap of the CPR. The design of the quarter-wave CPR includes a superconducting loop formed by the ground planes of the resonator (blue in Fig. 2 ). When a field perpendicular to the substrate is applied, such as the bias field, a screening current is induced in the ground planes and ensures the conservation of the magnetic flux in this superconducting loop. Such a current, that circulates just next to the gap, generates a magnetic field profile that guides the atoms into the gap. At distances comparable to the width of the ground planes, such guiding is further enhanced by the MOE that focuses magnetic field lines and generates magnetic gradients that centre the cloud in the gap. The guiding of atoms into the gap is observed by in situ measurements of the position of the atomic cloud for different bias field orientations (angle α in Fig. 3a ) and different currents in the wire ( Fig. 3a ). For each experimental point, the cloud is first brought to a trap-wire distance of ~100 μm, rotated to the angle α and then moved to the desired trapping current. The measured position ( y , z ) agrees well with a 2D simulation of the London equations [36] that includes gravity and the conservation of flux in the resonator loop (see Methods). The simulations are performed without free parameters. As experimentally observed and consistent with our model, we note that the two gaps of the CPR are not equivalent. Owing to the opposite direction of the current in the ground planes and the orientation of the bias field, only the closest gap to the trapping wire can be accessed. We call this trap, resulting from applied and induced currents, a hybrid trap. 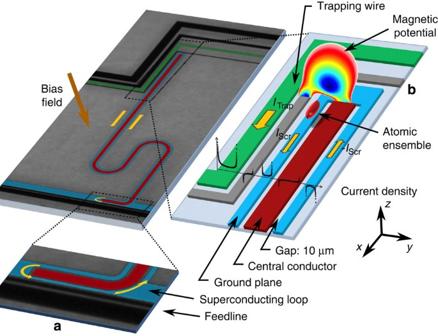Figure 2: Atom-trapping scheme. Scheme of the atoms trapped in the gap of a superconducting quarter wavelength coplanar microwave resonator (CPR). (a) Zoom of the superconducting link between the two ground planes of the CPR. (b) Zoom of the structure around the trapping region. The trap inside the gap is a result of the magnetic fields generated by the current of the trapping wireITrapand by the screening currentIScrin the ground plane. These fields cancel with an externally applied bias field. The embedded plot (black dots) is the simulated distribution of the screening currents in the superconductor. These currents keep the flux in the superconducting loop constant and the interior of the films field free. The transverse profile of the magnetic potential is shown in colour. The dark blue corresponds to the potential minimum. Figure 2: Atom-trapping scheme. Scheme of the atoms trapped in the gap of a superconducting quarter wavelength coplanar microwave resonator (CPR). ( a ) Zoom of the superconducting link between the two ground planes of the CPR. ( b ) Zoom of the structure around the trapping region. The trap inside the gap is a result of the magnetic fields generated by the current of the trapping wire I Trap and by the screening current I Scr in the ground plane. These fields cancel with an externally applied bias field. The embedded plot (black dots) is the simulated distribution of the screening currents in the superconductor. These currents keep the flux in the superconducting loop constant and the interior of the films field free. The transverse profile of the magnetic potential is shown in colour. The dark blue corresponds to the potential minimum. 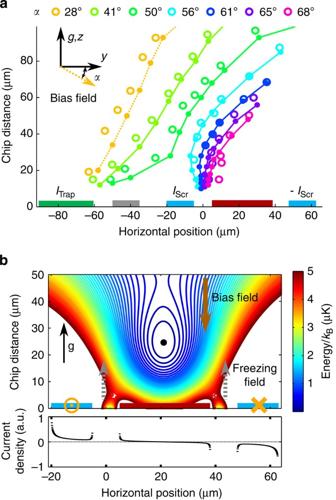Figure 3: Positioning atoms close to a superconducting coplanar microwave resonator. (a) Position of the trap for different currents in the trapping wire and different anglesαbetween the bias field and the surface of the chip.α=arctanis varied by changingwith=2.3 G constant. The position of the atoms has been measured byin situabsorption imaging (Methods). For small angles, the trap behaves as for a normal conducting chip, that is, when the current is reduced in the trapping wire (ITrap), the trap moves towards it. For large angles, this behaviour is modified and the trap is focused into the gap between the centre conductor and the ground plane of the CPR. The agreement between measurement (circles) and simulations (dotted and solid lines with dots) proves that positioning of the atoms in the gap of the CPR can be facilitated by screening currentsIScrin the ground planes. The simulations36are performed with no adjustable parameter and assume a Meissner state for the superconductor. Gravity,g, is oriented upwards. (b) Top: potential energy landscape of a persistent-current trap above the central conductor (red) of the CPR. This trap is generated by the superposition of a vertical homogeneous bias field≈1.2 G and the field induced by the screening currents. To enhance the screening currents at a given bias field, a non-zero flux is trapped in the gap of the CPR during the cool-down of the cryostat (freezing field,≈0.5 G). Isolines are separated by 100 nK. Bottom: screening current density distribution induced by the combination of bias field and freezing field. Full size image Figure 3: Positioning atoms close to a superconducting coplanar microwave resonator. ( a ) Position of the trap for different currents in the trapping wire and different angles α between the bias field and the surface of the chip. α =arctan is varied by changing with =2.3 G constant. The position of the atoms has been measured by in situ absorption imaging (Methods). For small angles, the trap behaves as for a normal conducting chip, that is, when the current is reduced in the trapping wire ( I Trap ), the trap moves towards it. For large angles, this behaviour is modified and the trap is focused into the gap between the centre conductor and the ground plane of the CPR. The agreement between measurement (circles) and simulations (dotted and solid lines with dots) proves that positioning of the atoms in the gap of the CPR can be facilitated by screening currents I Scr in the ground planes. The simulations [36] are performed with no adjustable parameter and assume a Meissner state for the superconductor. Gravity, g , is oriented upwards. ( b ) Top: potential energy landscape of a persistent-current trap above the central conductor (red) of the CPR. This trap is generated by the superposition of a vertical homogeneous bias field ≈1.2 G and the field induced by the screening currents. To enhance the screening currents at a given bias field, a non-zero flux is trapped in the gap of the CPR during the cool-down of the cryostat (freezing field, ≈0.5 G). Isolines are separated by 100 nK. Bottom: screening current density distribution induced by the combination of bias field and freezing field. Full size image A further advantage in using superconductors to manipulate cold atoms is the possibility to engineer traps induced by persistent currents. These persistent-current traps [14] render the direct injection of currents on the chip unnecessary and therefore suppress the related source of noise. In our geometry, such a trap can be generated directly below the CPR. Here we demonstrate a self-centred trap generated by a single homogeneous bias field and its induced screening currents. By trapping flux in the resonator loop with a freezing field applied during the cooling of the cryostat, the magnitude of the screening currents can be controlled independently from the applied bias field. This experimentally realized trap is simulated in Fig. 3b , where both the resulting potential and the current densities are depicted. The simulation presented includes the distortion due to the MOE, the conservation of magnetic flux in the loop and the effect of vortices trapped inside the film during the cooling of the cryostat [37] , [38] . The agreement of position and trap frequencies between the experiment and our simple model requires an adjustment of the input parameters by <20%. In the trap of Fig. 3b with oscillation frequencies {35, 173, 107} Hz, a cloud at T ~90 nK starting with >30% condensed fraction and a central density <8 × 10 13 at cm −3 has a lifetime of 10(4) s, probably limited by the shallow trap depth (~320 nK). We stress that, in this loop geometry, the conservation of magnetic flux should reduce the amplitude of external magnetic noise at the trap position. Coherence in a superconducting CPR To study the coherence lifetime of atomic ensembles in the close vicinity of a CPR, we perform Ramsey measurements at different positions below the superconducting chip. These measurements compare the coherence of a trapped atomic ensemble in a superposition of the states |0 =| F =1, m F =−1 and |1 =| F =2, m F =1 ( Fig. 1f ) with a high-stability 10 MHz reference oscillator that has a short- and long-term frequency stability Δ f / f <5 × 10 −12 . These two states are chosen for the low sensitivity of their transition frequency to magnetic inhomogeneities at a magnetic offset field of 3.228 G (see Methods) [39] . The atomic cloud is first prepared in a thermal and pure state of |0 . The initialization of the coherent superposition is realized by a π /2 two-photon excitation that starts the interferometric sequence. After a variable waiting time T R , the interferometer is closed by a second π /2 pulse. The populations N 0 ( T R ) and N 1 ( T R ) in, respectively, | F =1 and | F =2 are consecutively read out by state-selective absorption imaging (see Methods), and the resulting probability of | F =2 : N 1 ( T R )/( N 0 ( T R )+ N 1 ( T R )) is displayed in Fig. 4a–c . 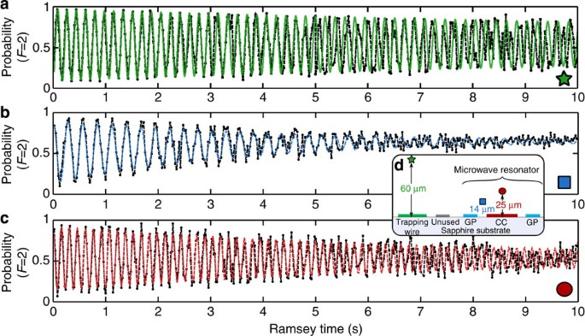Figure 4: Atomic coherence in a superconducting coplanar microwave resonator. Ramsey fringes measured in the time domain for different trapping positions on the superconducting atom chip. From top to bottom, the trapping positions correspond to: (a) the reference trap (green star in (d)), (b) the hybrid trap (blue square in (d)) and (c) the persistent-current trap (red disk in (d)). The coherence time obtained for the three sets are 20.5, 3.9 and 7.8 s, respectively, that indicate collision-induced SSR effects25(see main text and Methods). The coherence time of each set is estimated by measuring the fringe contrast decay on time intervals in which the phase is preserved. Black dots are experimental data and coloured lines are fits, with a fixed decay, to the first few seconds of the oscillation: 5, 3 and 4 s, respectively. Inset (d): positions of the different traps. The reference trap is situated 60 μm straight below the trapping wire. The hybrid trap, which is generated by applied and induced currents, stands 14 μm below the 10-μm-wide gap of the CPR. The persistent-current trap is 25 μm below the central conductor (CC) of the CPR that has a width of 33 μm. GP stands for ground planes. Horizontal and vertical axes are to scale. The experimental parameters for each measurement are summarized inTables 1and2. Figure 4: Atomic coherence in a superconducting coplanar microwave resonator. Ramsey fringes measured in the time domain for different trapping positions on the superconducting atom chip. From top to bottom, the trapping positions correspond to: ( a ) the reference trap (green star in ( d )), ( b ) the hybrid trap (blue square in ( d )) and ( c ) the persistent-current trap (red disk in ( d )). The coherence time obtained for the three sets are 20.5, 3.9 and 7.8 s, respectively, that indicate collision-induced SSR effects [25] (see main text and Methods). The coherence time of each set is estimated by measuring the fringe contrast decay on time intervals in which the phase is preserved. Black dots are experimental data and coloured lines are fits, with a fixed decay, to the first few seconds of the oscillation: 5, 3 and 4 s, respectively. Inset ( d ): positions of the different traps. The reference trap is situated 60 μm straight below the trapping wire. The hybrid trap, which is generated by applied and induced currents, stands 14 μm below the 10-μm-wide gap of the CPR. The persistent-current trap is 25 μm below the central conductor (CC) of the CPR that has a width of 33 μm. GP stands for ground planes. Horizontal and vertical axes are to scale. The experimental parameters for each measurement are summarized in Tables 1 and 2 . Full size image To study the capabilities of our setup, we first describe a reference measurement that is performed far from the CPR: 60 μm below the third trapping wire (green star: Fig. 4a ). This measurement is conducted with 1.9(4) × 10 4 atoms at a temperature of 245(30) nK in a magnetic trap with oscillation frequencies {10, 215, 181} Hz, corresponding to a mean density (in units of 10 12 at/cm 3 ) ≈0.4(1). In this configuration, the coherence time, as measured by the decay of the envelope, is T coh =20.5(6.0) s (1/ e exponential decay time). Owing to magnetic noise in this non-shielded apparatus and drifts over the length of the scan (several hours), the phase starts to be lost for T R >5 s, corresponding to a technically induced reduction of the T 2 time of the ensemble. The observed decay time T coh exceeds the time of 6 s predicted by the residual trap inhomogeneities Δ 0 /2 π ≈0.04 Hz (see Methods [40] ). This indicates that we entered the spin self-rephasing (SSR) regime [25] , where the identical spin rotation rate ω ex /2 π =3 Hz dominates both Δ 0 and the rate of lateral elastic collisions γ c =1 s −1 . This regime can be understood as a continuous spin-echo process triggered by forward atomic collisions. The second trap under study is the hybrid trap, situated 14 μm below the gap of the CPR. As mentioned before, this position is particularly privileged for the perspective of strong atom–cavity coupling. The Ramsey fringes shown by blue squares ( Fig. 4b ) were obtained for 1.25(40) × 10 4 atoms at a temperature of 320(20) nK held in a confined trap {16. 9, 451, 390} Hz, corresponding to ≈1.24(40). The coherence time is T 2 ≈ T coh =3.9(5) s. The reduction with respect to the reference position is mainly explained based on the atom loss decay time of 3.4(2) s of the hybrid trap. This loss rate is asymmetric and mainly affects the state |1 . It is partially explained by spin-exchanging collisions that transfer two collisioning atoms in |1 towards the states | F =2, m F =0 (untrapped) and | F =2, m F =2 (trapped). In Fig. 4b , this collision process is responsible for the asymmetry of the probability for large T R . It comes as a drawback of the guiding mechanism that strongly compresses the trap and increases the atomic density (see Table 1 ). The spin-exchanging collision rate γ 22 =1.6 × 10 −13 cm 3 s −1 reported in Egorov et al. [41] is insufficient to fully explain our observed loss rate and other possible mechanisms are under study. The fringes presented in Fig. 4b result from an optimization of the temperature that is high enough to minimize collisional losses and low enough to enter the SSR regime ( ω ex /2 π =9.5 Hz, γ c =3.6 s −1 , Δ 0 /2 π =0.12 Hz). Table 1 Results of atomic coherence. Full size table The last position studied corresponds to the persistent-current trap previously mentioned (red disk: Fig. 4c ). In this trap the measurement was performed with 1.25(40) × 10 4 atoms at 158(23) nK, corresponding to ≈0.78(30) and to the related SSR parameters ω ex /2 π =6 Hz, γ c =1.6 s −1 and Δ 0 /2 π =0.1 Hz. The coherence lifetime obtained is T 2 ≈ T coh =7.8(14) s and is mainly limited, in this shallow trap (~320 nK), by the atom loss decay time 4.8(3) s. The three measurements are compared in Table 1 . It shows that the trap deformation induced by the superconducting CPR results in an increase in the trap frequencies, which impact the coherence of the atomic cloud. We do not expect that such coherence would change for a cavity on-resonance with the transition from |0 to |1 that necessarily involves two photons. Nevertheless, thermal photons in a cavity that would be on resonance with one of the transitions from |0 or |1 to untrapped states could open an asymmetric loss channel and a corresponding loss of coherence. In the effective strong coupling limit that we target, this process could be used to cool the mode of the resonator [20] . In conclusion, we have demonstrated that, in the vicinity of a superconducting CPR, magnetic traps can be engineered to produce robust and controllable conditions for the coherent manipulation of atoms. The preparation of large BECs and thermal clouds of a million atoms opens the path to the strong collective coupling to a CPR, and to the transfer of quantum information between atomic and superconducting systems. The long coherence of atomic superposition states on the time scale of seconds encourages the development of cold atom/superconductor hybrid quantum systems in which cold atoms would serve as quantum memory. Although the motion of particles is usually considered as a source of decoherence, which, for example, prevents the use of spin-echo techniques, it has an important role in this experiment to maintain the coherence of the superposition state. If such a mechanism can be extended to preserve the coherence of single excitations, it will surely lead to very rich dynamics of collective states. Atom cloud preparation The magneto-optical trap (MOT) is loaded from a 2D-MOT. For a loading time of 6 s, the MOT contains ~10 9 87 Rb atoms at a temperature of ~200 μK. With this method, we do not observe perturbation of the background pressure. After an optical molasses, the atomic cloud is optically pumped into one of the two hyperfine ground states |0 or | F =2, m F =2 (total angular momentum states) and is transferred through a magnetic quadrupole into a harmonic Ioffe−Pritchard-type trap. It is further cooled by forced RF evaporation to a temperature of ~1.5 μK, slightly above the BEC transition. The remaining 5 × 10 6 atoms are loaded into optical tweezers ( λ =1064, nm laser, P =500 mW, focused to w 0 =25 μm beam waist) and transported without significant loss or heating over a distance of 40 mm to the superconducting chip. During the optical transfer, a quantization field of 350 mG along x is applied to maintain the polarization of the sample. Magnetic field calibration At the position of the atomic cloud, below the superconducting chip, the magnetic field is controlled by three orthogonal pairs of coils that allow to independently control the three directions of space. The calibration of the residual field and the field generated by the coils is realized in situ by microwave spectroscopy. To that purpose, the atoms are prepared in |0 and the magnetic field is set to the desired field of study. After all Eddy currents have damped out, the atoms are released from the optical dipole trap. The microwave transition considered is |0 to | F =2, m F =0 . In the absence of a magnetic field it has a frequency of 6.834682610 GHz and a first-order Zeeman sensitivity of 700 kHz G −1 . In a first coarse step, the absolute field is reduced to below 5 mG. In a second fine step, each pair of coils is switched on in a row to generate a frequency shift of approximately 200 kHz. This shift is then measured with an accuracy of ±500 Hz. This way, each pair of coils is in situ and independently calibrated (residual contribution from other pairs below 1%) and the residual field is measured to below 1 mG, while the coils are calibrated with an accuracy better than 0.3%. To avoid perturbation by the MOE of the nearby superconductor, this calibration is done with the cryostat at T ≈10 K. Imaging and measurement of position The atoms are observed by absorption imaging with a variable time of flight (TOF). The large BEC in Fig. 1d was measured by off-resonance imaging, which was calibrated on a low-density cloud. Owing to eddy currents in the mechanical system, the measured atom number is not absolute and depends on the TOF. For TOF<10 ms, the calibration of the detection of the state |0 with respect to the state |1 is obtained by minimizing the variance of the total atom number detected over the length of the scan. For TOF>10 ms, atom numbers stay constant, showing that eddy currents are no more an issue at the corresponding distances. The absolute calibration of the atom number is obtained from the critical temperature of Bose−Einstein condensation. This calibration is the main source of uncertainty of the atom numbers (20%). Therefore, the atom number uncertainty quoted in the text does not represent shot-to-shot fluctuations. The state-selective measurement realized for the coherence measurement is done by first measuring and blasting the atoms in F =2, and second by repumping and measuring the atoms in F =1. The two measurements are realized on orthogonal axes. In situ , the position of the atomic cloud is measured along the three directions of space by two reflection imaging systems that are aligned along x and y . The calibration of distances is realized by TOF of the magnetically insensitive state | F =2, m F =0 . To avoid spurious effects, the chip is uncoated. Magnetic field calculations To calculate the current densities in the superconductor and the subsequent atomic trap deformation, we solved the London equations using the 2D algorithm described in Cano et al. [36] This treatment is particularly valid in the trapping region where thin films are parallel to each other. The assumption of a pure Meissner state can be justified by an estimate of the maximum fields at the lead edges [42] . In our field and current range, these edge fields remain considerably below the lower critical field of a dirty niobium film [43] , assuming a penetration depth λ L ≈100 nm and a Ginzburg−Landau parameter κ ≈10. The conservation of flux in the superconducting loop of the resonator is further taken into account by imposing net currents in the grounds of the resonator. The influence of an homogeneous density of vortices pointing along z is modelled by the superposition of an homogeneous field along z (undeformed) and the opposite field deformed by the superconducting structure in a pure Meissner state. In all simulations, the quantization of flux is neglected (Φ 0 /Φ≈5 × 10 −5 ). The simulations presented in Figs 2 and 3 have been confirmed using a 3D simulator (3D-MLSI [44] ). The effect of gravity is included in all simulations. Details on the measurement of coherence lifetime The measurement of the T coh time of the atomic qubit formed by the state |0 and |1 is realized by a Ramsey-type experiment. As shown in Fig. 1f , the two states are coupled via a two-photon transition involving a microwave photon at f MW =6.83337816 GHz and an RF photon at f RF =1.3 MHz. Both frequencies are generated by commercial synthesizer phase locked to a high-stability 10 MHz quartz oscillator (Oscilloquartz, 8607-BHM15), and their sum is frequency detuned from the atomic transition by Δ R /2 π . For all the measurement presented, the microwave with power P MW is radiated by an helicoidal antenna situated outside the vacuum chamber at a distance of 20 cm from the atoms. The RF with power P RF is coupled on the chip to the largest Z -wire. The Rabi frequency Ω R obtained in each situation is summarized in Table 2 . 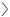Figure 5: Differential frequency shift of the |0to |1transition. The black points are experimental data. The red dashed line is the prediction given by the Breit–Rabi formula45. Figure 5 shows the differential frequency shift of the qubit transition that is well approximated by Δ ν ( r )= ν |1› − ν |0› =Δ ν 0 + β ( B ( r )− B 0 ) 2 , with Δ ν 0 =4.4973, kHz, B 0 =3.228917(3) G (ref. 25 ) and β =431.36 Hz/G 2 (ref. 39 ). At the magic offset field B 0 , this shift is first-order insensitive to the magnetic field. The sensitivity of the coherence time to the magnetic inhomogeneities of the trap is therefore highly reduced. The measurements presented in Fig. 4 are performed with an offset field B off slightly lower than B 0 . This configuration is known as the mutual compensation scheme [39] , [40] , which allows to compensate the negative collisional shift Δ c ( r )/2 π =−0.4 n ( r )/10 12 Hz by the positive magnetic shift Δ B ( r )=2 π Δν( r ). In such conditions, an optimum residual radial frequency homogeneity Δ 0 = is obtained for an optimal offset field that depends on the number of particles, the temperature and the geometry of the trap. In Table 2 , we give the optimum value of Δ 0 for each experimental configuration. In the abscence of spin-rephasing, such inhomogeneities should result in a decay of the Ramsey contrast with a time constant τ inh = /Δ 0 (ref. 40 ). Table 2 Experimental parameters for atomic coherence measurements. Full size table Figure 5: Differential frequency shift of the |0 to |1 transition. The black points are experimental data. The red dashed line is the prediction given by the Breit–Rabi formula [45] . Full size image How to cite this article: Bernon, S. et al. Manipulation and coherence of ultra-cold atoms on a superconducting atom chip. Nat. Commun. 4:2380 doi: 10.1038/ncomms3380 (2013).